Solution-processed multilayer small-molecule light-emitting devices with high-efficiency white-light emission Recent developments in the field of π-conjugated polymers have led to considerable improvements in the performance of solution-processed organic light-emitting devices (OLEDs). However, further improving efficiency is still required to compete with other traditional light sources. Here we demonstrate efficient solution-processed multilayer OLEDs using small molecules. On the basis of estimates from a solvent resistance test of small host molecules, we demonstrate that covalent dimerization or trimerization instead of polymerization can afford conventional small host molecules sufficient resistance to alcohols used for processing upper layers. This allows us to construct multilayer OLEDs through subsequent solution-processing steps, achieving record-high power efficiencies of 36, 52 and 34 lm W −1 at 100 cd m −2 for solution-processed blue, green and white OLEDs, respectively, with stable electroluminescence spectra under varying current density. We also show that the composition at the resulting interface of solution-processed layers is a critical factor in determining device performance. Current organic light-emitting devices (OLEDs) typically consist of four or more multiple layers of different materials in precise opto-electrical design. Such multilayer structures allow for the separation of the charge-injecting, charge-transporting and light-emitting functions to the different layers, thus leading to a marked increase in efficiency and lifetime [1] , [2] , [3] , [4] , [5] . Although stepwise vacuum evaporation easily achieves the required multilayer structures of small molecules at the expense of high manufacturing cost, it is more challenging in the case of solution processing, because depositing one layer would dissolve the layer beneath it. To achieve the multilayer structures by solution processing, research efforts have focused on π-conjugated polymers that afford a robust hydrophobic layer, on which a hydrophilic layer can be deposited from orthogonal solvents, such as water or water/alcohol mixture [6] , [7] , [8] , [9] , [10] . In situ cross-linking reactions have also been explored to afford covalently bound structures that are highly resistant to processing solvents [11] , [12] , [13] , [14] , [15] , [16] , [17] , [18] , [19] . Despite their high mechanical robustness and compatibility with subsequent solution processing, polymers are plagued by limited reproducibility in the device performance because of batch-to-batch variations with respect to molecular weight, polydispersity, regioregularity and purity [20] , [21] , [22] , [23] . Moreover, their efficiencies are still far below the fluorescent tubes [24] . Thus far, the highest reported power efficiency of white polymer LEDs is ~25 lm W −1 (refs 7 , 25 ). On the other hand, small molecules are very attractive because they have a well-defined molecular structure that offers more reproducibility of synthesis procedures and better understanding of molecular structure–device performance relationships. However, their thin-film assemblies, most of which are amorphous in nature, are easily broken up, even by the orthogonal solvents, because small molecules typically attach to each other only by weak intermolecular forces such as van der Waals, H-bonding and π–π stacking interactions. Consequently, the highest reported efficiency of solution-processed small-molecule OLEDs still relies on a vacuum-evaporated electron-transporting layer (ETL), which is not practical for low-cost mass production of scalable devices [26] . Herein, we demonstrate highly efficient small-molecule OLEDs in which quadruple organic layers, including a molecular-emitting layer (EML) and ETL, are fully solution processed. The key feature of the devices is the use of newly developed small host molecules in the EML, which are sufficiently resistant to the orthogonal solvents such as alcohols, used for processing upper ETLs, thus allowing us to construct the multilayer structure through subsequent solution-processing steps. While a robust host polymer is typically required to realize the multilayer structure, we simply modified conventional host molecules by covalent dimerization or trimerization to afford sufficient resistance to alcohols. With this approach, record-high efficiencies have been achieved for solution-processed blue, green and white OLEDs. Solvent resistance test Through experiments with 17 host molecules over a wide range of molecular weight from 243–1,146 ( Fig. 1a ), we found that their resistance to alcohols remarkably increases with molecular weight. 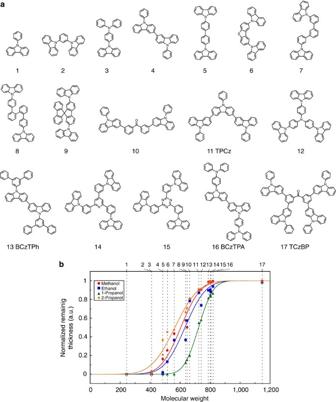Figure 1: Solvent resistance of molecular thin films. (a) Molecular structures of the host molecules arranged in order of increasing molecular weight. (b) Plots of normalized remaining thickness of the molecular thin films after rinsing with a variety of alcohols as a function of molecular weight. The solid lines represent the best fit to the cumulative distribution function. Figure 1b shows the normalized remaining thickness of molecular thin films after rinsing with a variety of alcohols as a function of molecular weight, as measured by ultraviolet–visible absorption spectroscopy. From the best-fit cumulative distribution function, we determined that the threshold molecular weights for achieving 95% remaining thickness were 775, 811, 849 and 767 μ for methanol, ethanol, 1-propanol and 2-propanol, respectively. This result demonstrates that even conventional host molecules can be compatible with the subsequent solution process simply by covalent dimerization or trimerization to exceed the threshold molecular weights, eliminating the need for polymeric counterparts. In addition, this figure covers a wide variety of building blocks, including arene, carbazole, triphenylamine, fluorene, benzothiophene and even polar moieties such as benzophenone, pyridine and triazine, making this approach broadly applicable. We also note that our approach enables subsequent solution processing onto the EML without having to use water, which is detrimental to device efficiency and stability [27] , [28] , [29] , [30] . Figure 1: Solvent resistance of molecular thin films. ( a ) Molecular structures of the host molecules arranged in order of increasing molecular weight. ( b ) Plots of normalized remaining thickness of the molecular thin films after rinsing with a variety of alcohols as a function of molecular weight. The solid lines represent the best fit to the cumulative distribution function. Full size image Solution-processed green OLEDs On the basis of the above estimates, we elected to use two host molecules for green phosphorescent OLEDs: 3,3′:6′,3′′-ter(9-phenyl-9 H-carbazole) (11, TPCz) and 3,3′,6,6′-tetrakis(9-phenyl-9 H-carbazol-3-yl)benzophenone (17, TCzBP). The synthesis and characterization details for the host molecules can be found in the Supplementary Information . The schematic energy diagram of the host molecules is shown in Fig. 2b . When mixing the two host molecules in an EML, holes should preferentially reside in the shallow highest-occupied molecular orbital of TPCz and electrons in the deep lowest-unoccupied molecular orbital of TCzBP. Consequently, we can accurately optimize charge balance in the device by varying the ratio of the two host molecules to achieve high efficiency. 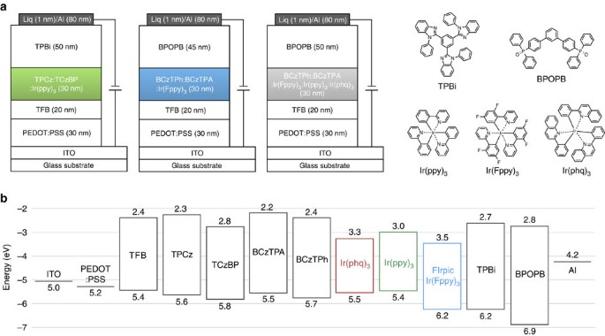Figure 2: Device structure of the solution-processed OLEDs. (a) Schematic of the optimized device and molecular structures of the materials used. (b) Schematic energy-level diagram of the materials. Figure 2: Device structure of the solution-processed OLEDs. ( a ) Schematic of the optimized device and molecular structures of the materials used. ( b ) Schematic energy-level diagram of the materials. Full size image By using the two molecules as hosts for tris(2-phenylpyridine)iridium(III) (Ir(ppy) 3 ), we fabricated green phosphorescent OLEDs, in which quadruple organic layers were fully solution processed. The device configuration was indium tin oxide (ITO) (130 nm)/poly(3,4-ethylenedioxythiophene):poly(styrenesulfonate) (PEDOT:PSS) (30 nm)/poly(9,9-dioctyl-fluorene- alt - N -(4-butylphenyl)-diphenylamine) (TFB) (20 nm)/host:12 wt% Ir(ppy) 3 (30 nm)/2,2′,2′′-(1,3,5-benzinetriyl)tris(1-phenyl-1-H-benzimidazole) (TPBi) (50 nm)/lithium 8-quinolate (Liq) (1 nm)/Al (100 nm) ( Fig. 2a ). In these devices, TPBi was elected as an ETL because of its sufficient solubility in methanol, enabling the subsequent solution processing on the molecular EML. The most common host polymer poly( N -vinylcarbazole) (PVK) was also used for comparison. By mixing a 1:1 ratio of TPCz and TCzBP, we achieved a power efficiency of 52 lm W −1 at 100 cd m −2 . Indeed, the peak power efficiency reached an extremely high value of 96 lm W −1 . The corresponding external quantum efficiency (EQE) was 23%, which remained as high as 22 and 20% at 100 cd m −2 and 1,000 cd m −2 , respectively ( Fig. 3a,b , Supplementary Table 1 ). These efficiencies are considerably higher than those of the PVK based device and the best polymer light-emitting diodes ever reported in the literature [11] and even comparable with those of evaporated multilayer OLEDs [31] . We also note that there is no perceivable change in luminance as a function of viewing angle (Lambertian factor: 1.03), eliminating the possibility of overestimating the efficiencies. 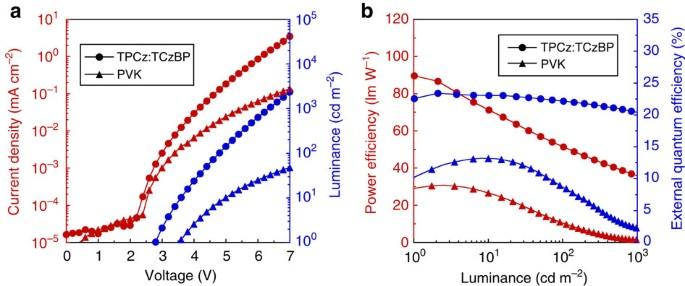Figure 3: Device performance of the green OLEDs. (a) Current density−voltage, luminance−voltage (b) power efficiency−luminance and EQE−luminance characteristics. Figure 3: Device performance of the green OLEDs. ( a ) Current density−voltage, luminance−voltage ( b ) power efficiency−luminance and EQE−luminance characteristics. Full size image Solution-processed blue OLEDs Despite the impressive efficiencies of the green phosphorescent OLEDs, our initial attempt at using standard blue phosphorescent emitter bis(2-(4,6-difluorophenyl)pyridine) (picolinate)iridium(III) (FIrpic) resulted in poor efficiencies. In the blue OLEDs, 4,4′-(3,3′-bi(9 H-carbazole)-9,9′-diyl)bis(2,6-diphenyl) benzene (13, BCzTPh) and 4,4′-(3,3′-bi(9 H-carbazole)-9,9′-diyl)bis( N,N -diphenyl)aniline (16, BCzTPA) were employed as host molecules and 2-propanol-soluble 1,3-bis(3-(diphenylphosphoryl)phenyl)benzene (BPOPB) was used as an ETL. The device configuration was ITO (130 nm)/PEDOT:PSS (30 nm)/TFB (20 nm)/host:12 wt% FIrpic (30 nm)/BPOPB (45 nm)/Liq (1 nm)/Al (100 nm) ( Fig. 2a ). While these host molecules have a sufficiently high triplet energy level ( T 1 ) for efficient exothermic energy transfer to the phosphorescent blue emitter ( Supplementary Table 2 ), the resulting device exhibited considerable emission from the host molecules at around 420 nm ( Fig. 4a ) and a low power efficiency of 6.5 lm W −1 at 100 cd m −2 ( Fig. 4c ). Alternatively, with three-coordinated tris(2-(4,6-difluorophenyl)pyridine)iridium(III) (Ir(Fppy) 3 ), the device efficiencies significantly increased to 36 lm W −1 for power efficiency and 20% for EQE at 100 cd m −2 ( Fig. 4c , Supplementary Table 1 ). 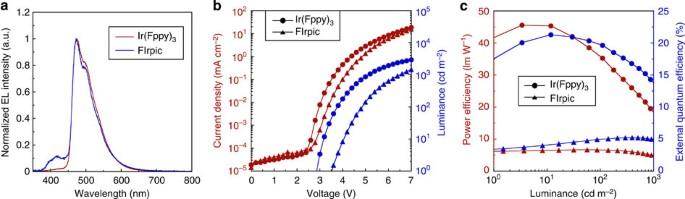Figure 4: Device performance of the blue OLEDs. (a) EL spectra, (b) current density−voltage, luminance−voltage (c) power efficiency−luminance and EQE–luminance characteristics. Figure 4: Device performance of the blue OLEDs. ( a ) EL spectra, ( b ) current density−voltage, luminance−voltage ( c ) power efficiency−luminance and EQE–luminance characteristics. Full size image It is intriguing to note that Ir(Fppy) 3 performs five times as well as FIrpic in power efficiency, although these two blue emitters possess almost identical opto-electrical properties ( Supplementary Table 2 ). In these devices, the majority of excitons would be generated near the EML/ETL interface because of the relatively large injection barrier between them ( Fig. 2b ), and would subsequently be harvested by the doped blue phosphorescent emitter. In addition, we have previously reported that the direct electron-trapping process of a blue phosphorescent emitter played a major rule in efficient electron injection at the EML/ETL interface in evaporated OLEDs [32] . We thus hypothesized that polar picolinate ligand-containing FIrpic would dissolve away from the EML surface upon the subsequent solution processing of the ETL from the 2-propanol solution, resulting in the unwanted host emission and poor device efficiencies. Depth-profiling analysis To verify the hypothesis, we performed depth-profiling measurements of the devices by time-of-flight secondary ion mass spectrometry (TOF-SIMS). These measurements involved Ar 2500 + gas cluster ion beam etching [33] starting from the ETL surfaces to the underlying substrates. This direction of etching allows for collecting the composition of the EMLs without alternating their original position at the EML/ETL interfaces (peak fronts), while etching and primary ion beams cause peak tailing. 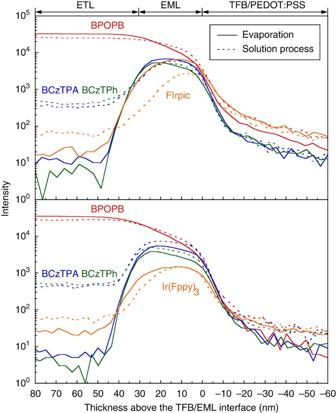Figure 5: TOF-SIMS depth profiles of the blue OLEDs with different emitters. The dashed lines represent depth profiles of the devices using solution-processed ETLs. The solid lines represent data for reference devices using evaporated ETLs. Figure 5 displays the TOF-SIMS depth profiles of the solution-processed devices with the different blue phosphorescent emitters, FIrpic and Ir(Fppy) 3 , in comparison with reference devices with a vacuum-evaporated ETL, for which a well-defined interface is expected to exist between the EML and ETL. We focused on [C 22 H 12 F 4 IrN 2 ] + ions with m/z =573 as signatures both of FIrpic and Ir(Fppy) 3 to obtain sufficient intensity in the dilute emitters embedded in the host matrix. We also monitored the corresponding molecular ions for the other molecules. The depth resolution was 11.5 nm under our experimental conditions. Figure 5: TOF-SIMS depth profiles of the blue OLEDs with different emitters. The dashed lines represent depth profiles of the devices using solution-processed ETLs. The solid lines represent data for reference devices using evaporated ETLs. Full size image One observed form the TOF-SIMS depth profiles that the composition at the solution-processed EML/ETL interface was significantly varied between the FIrpic and Ir(Fppy) 3 system. Ir(Fppy) 3 showed a slight reduction in intensity in the interface region of roughly 10–20 nm for the solution-processed device, whereas a noticeable reduction in FIrpic intensity occurred almost over the entire EML, particularly at the EML/ETL interface. The corresponding reduction in the concentration of the blue emitters was also quantitatively observed by high-performance liquid chromatography analysis ( Supplementary Fig. 1 ); the reduction in concentration of emitters was 48% and 8% for FIrpic and Ir(Fppy) 3 , respectively, upon rinsing with pure 2-propanol. These results indicate that almost half of the FIrpic molecules dissolved from the EML while depositing the ETL, and the host molecules were compositionally rich in the resulting interface. On the other hand, the Ir(Fppy) 3 molecules existed over the entire EML, including the interface even after the deposition of the ETL. The improved device efficiencies upon introduction of Ir(Fppy) 3 therefore arise from the efficient electron injection at the EML/ETL interface through the direct electron-trapping process of Ir(Fppy) 3 . We also note that a very small amount of the EML composition migrated and uniformly distributed into the solution-processed ETL. Solution-processed white OLEDs Finally, we fabricated solution-processed multilayer white OLEDs by incorporating green-emitting Ir(ppy) 3 (0.2 wt%) and red-emitting tris(2-phenyl-1-quinoline)iridium(III) (Ir(phq) 3 ) (0.7 wt%) into the blue EML. Although the electroluminescence (EL) spectra of white OLEDs typically depend on current density (in other words, luminance) [4] , [6] , [19] , [34] , [35] , [36] , [37] , the resulting solution-processed white OLED surprisingly showed no perceived change in the EL spectra under varying current density, as shown in Fig. 6a . The corresponding colour shift in the Commission Internationale de l'éclairage (CIE) coordinates was as small as Δx , y =0.002, 0.002 between 100 and 1,000 cd m −2 . For comparison, the evaporated ETL exhibited relatively strong green and red emissions and a gradual blue shift in the CIE coordinates of Δx , y =0.054, 0.002 between 100 and 1,000 cd m −2 . 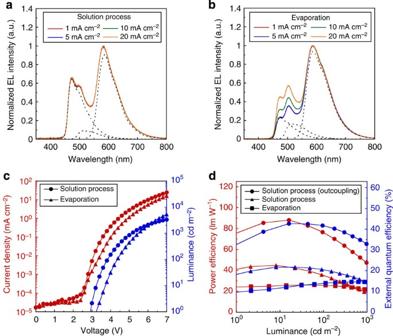Figure 6: Device performance of the white OLEDs. (a,b) EL spectra of the white OLEDs with the solution-processed ETL and the evaporated ETL under varying current density. The dashed lines represent the contributions of the three emitters determined by spectral fitting of the EL spectra at 1.0 mA cm−2. (c) Current density−voltage, luminance−voltage (d) power efficiency−luminance and EQE−luminance characteristics, for the white OLEDs. Figure 6: Device performance of the white OLEDs. ( a , b ) EL spectra of the white OLEDs with the solution-processed ETL and the evaporated ETL under varying current density. The dashed lines represent the contributions of the three emitters determined by spectral fitting of the EL spectra at 1.0 mA cm −2 . ( c ) Current density−voltage, luminance−voltage ( d ) power efficiency−luminance and EQE−luminance characteristics, for the white OLEDs. Full size image The stable EL spectra can be explained if the green and red emitters were partially washed away from the EML surface upon the solution processing of the ETL, causing electron trapping and recombination preferentially on the blue emitter at the EML/ETL interface. This would provide uniform exciton distribution among the three emitters, and thus the stable EL spectra, because the only exciton generation path left for the green and red emitters is energy transfer from the blue emitter staying at the EML/ETL interface. This hypothesis was confirmed with photoluminescence spectroscopy, showing that the red and green emissions of the EML decreased upon rinsing with pure 2-propanol ( Supplementary Fig. 2 ). Similar stable EL spectra have also been observed in evaporated OLEDs, in which the blue emitter is placed at the recombination interface and spatially separated from other emitters as in this case [2] . Figure 6d and Supplementary Table 1 summarize the efficiencies of the solution-processed white OLEDs. Remarkably, we achieved a high power efficiency of 34 lm W −1 and an EQE of 21% at 100 cd m −2 for a white emission with a colour rendering index of 70 and CIE coordinates of 0.43, 0.43 without the use of any outcoupling enhancement. The peak power efficiency and EQE reached 45 lm W −1 and 22%, respectively. To the best of our knowledge, these efficiencies are considerably higher than the highest efficiencies ever reported for white polymer LEDs [7] , [25] . In addition, when outcoupling all the photons trapped in the glass substrate, these efficiencies increase by a factor of 1.96 as confirmed by using an index-matched hemisphere lens. As a result, the maximum achievable power efficiency and EQE are expected to be 88 lm W −1 and 41%, respectively. We also note that the solution-processed device showed lower driving voltages and higher efficiencies compared with the corresponding device with an evaporated ETL ( Fig. 6c,d ). The superior performance with a solution-processed ETL was also observed in the green phosphorescent OLEDs using TPBi as an ETL ( Supplementary Fig. 3 ). To further understand the reason for the superior performance of the solution-processed devices, detailed studies of the electron-transporting properties of the solution-processed ETLs are currently underway. Materials Preparation and characterization of the materials used in this study can be found in Supplementary Methods . Solvent resistance testing Thin films of the host molecules were deposited by spin-casting from a tetrahydrofuran solution onto a 300-mm-diameter quartz disc to yield a film thickness of 30 nm, confirmed using a Dektak 8-surface profilometer. The thickness variation was monitored using a Shimadzu UV-3150 UV-vis-NIR spectrometer before and after spin-rinsing with 0.5 μl of alcohols such as methanol, ethanol, 1-propanol and 2-propanol. TOF-SIMS depth profiling The chemical composition of the surface was characterized using a PHI TRIFT V nanoTOF time-of-flight secondary ion mass spectrometer with a Au 3 ++ primary ion source operated at 30 kV, 9.0 nA and rastered over an area of 0.1 × 0.1 mm. Depth profiling was accomplished using the instrument’s Ar 2500 + ion source operated at 5 kV, 3.0 nA and rastered over 0.5 × 0.5 mm 2 . The depth resolution was determined using a procedure described by Shard et al . [38] OLED fabrication OLEDs were fabricated on glass substrates covered with ITO (sheet resistance of 10 Ω per square). The ITO substrates were ultrasonically cleaned with deionized water, acetone and 2-propanol, followed by ultraviolet–ozone treatment for 20 min. A 0.45-μm-filtered dispersion of PEDOT:PSS in water (Clevious P CH8000) was spin-cast onto the ITO substrate and then annealed at 200 °C for 10 min in ambient conditions to yield a 30-nm-thick thin film. After the annealing of PEDOT:PSS, all processes were performed under inert conditions. A solution of TFB in p -xylene at a concentration of 7.0 mg ml −1 was spin-cast onto PEDOT:PSS and then annealed at 200 °C for 60 min to yield a 20-nm-thick film insoluble in common organic solvents [39] , [40] . For the fabrication of the green OLEDs, a blend of TCzBP, TPCz and Ir(ppy) 3 in a tetrahydrofuran solution at a concentration of 5.5 mg ml −1 was spin-cast onto the TFB layer and then annealed at 150 °C for 30 min to yield the green EML, with a thickness of 30 nm. A solution of TPBi in methanol at a concentration of 6.7 mg ml −1 was spin-cast onto the EML and then annealed at 150 °C for 30 min to yield the ETL, with a thickness of 50 nm. For the fabrication of the blue and white OLEDs, a blend of BCzTPA, BCzTPh and the corresponding emitters in a tetrahydrofuran solution at a concentration of 5.0 mg ml −1 was spin-cast onto the TFB layer and then annealed at 100 °C for 10 min to yield blue and white EMLs, with a thickness of 30 nm. A solution of BPOPB in a 2-propanol solution at a concentration of 7.0 mg ml −1 was spin-cast onto the EML and then annealed at 70 °C for 10 min to yield the ETL, with a thickness of 45 nm and 50 nm for blue and white OLEDs, respectively. The cathode, consisting of a 1-nm-thick ultrathin Liq interfacial layer and a 100-nm-thick Al layer, was deposited by thermal evaporation at a base pressure of 1 × 10 −4 Pa. OLEDs were ready for characterization after encapsulation using an epoxy glue and a glass cover. OLED characterization All measurements were conducted in ambient air. The active area of each device was 2.0 × 2.0 mm 2 . Current–voltage characteristics were measured using a Keithley 2400 source meter. Luminance–voltage characteristics were measured using a Minolta CS-200 chromameter. EL spectra were measured using a Hamamatsu PMA-11 photonic multichannel analyzer. The angular dependence of the EL intensity was measured with a calibrated custom-built spectrogoniometer. The lens-based structure used to outcouple the light trapped in the substrate modes was a 30-mm-diameter half-sphere lens and was mounted on the substrate using an index-matching gel ( n =1.5). How to cite this article: Aizawa, N. et al . Solution-processed multilayer small-molecule light-emitting devices with high-efficiency white-light emission. Nat. Commun. 5:5756 doi: 10.1038/ncomms6756 (2014).